Probing charge screening dynamics and electrochemical processes at the solid–liquid interface with electrochemical force microscopy The presence of mobile ions complicates the implementation of voltage-modulated scanning probe microscopy techniques such as Kelvin probe force microscopy (KPFM). Overcoming this technical hurdle, however, provides a unique opportunity to probe ion dynamics and electrochemical processes in liquid environments and the possibility to unravel the underlying mechanisms behind important processes at the solid–liquid interface, including adsorption, electron transfer and electrocatalysis. Here we describe the development and implementation of electrochemical force microscopy (EcFM) to probe local bias- and time-resolved ion dynamics and electrochemical processes at the solid–liquid interface. Using EcFM, we demonstrate contact potential difference measurements, consistent with the principles of open-loop KPFM operation. We also demonstrate that EcFM can be used to investigate charge screening mechanisms and electrochemical reactions in the probe–sample junction. We further establish EcFM as a force-based imaging mode, allowing visualization of the spatial variability of sample-dependent local electrochemical properties. Understanding local electrostatic and electrochemical phenomena at the solid–liquid interface is crucial to areas ranging from corrosion [1] , [2] , sensing [3] , energy conversion [4] and storage [4] , [5] to biology and biochemistry [6] . Of particular interest are the local electrochemical processes governing the operation of energy conversion and storage devices, such as lithium ion batteries [7] , electrochemical capacitors [8] and fuel cells [9] . Significant progress has been achieved in developing a theoretical understanding of the complex diffuse-charge dynamics in electrochemical systems, involving both Faradaic (for example, redox reaction) and non-Faradaic (for example, electric double-layer charging) processes [10] , [11] , [12] , [13] . However, a complete understanding of such processes requires scanning probe microscopy (SPM) techniques capable of mapping electrostatic and electrochemical phenomena at the solid–liquid interface with a lateral resolution commensurate with the length scale of the phenomena. In ambient and vacuum environments, the electrostatic properties of surfaces can be mapped by Kelvin probe force microscopy (KPFM) [14] , [15] , [16] . In KPFM, the electrostatic force, F el =−½ C′ z ( V tip – V cpd ) 2 , acting on a probe due to the application of a tip voltage, V tip =V dc +V ac sin( ωt ), is detected via the first harmonic electrostatic force response of the cantilever, F ω =− C′ z ( V dc – V cpd ) V ac sin( ωt ), where V ac and V dc are AC voltage and DC bias applied to the tip (or sample), C′ z is the tip–sample capacitance gradient and V cpd is the contact potential difference (CPD) [14] . A feedback loop is employed to minimize the first harmonic response through the application of a DC bias proportional to the CPD between the probe and sample. The second harmonic component of the electrostatic force, F 2 ω =¼ C′ z V ac 2 cos(2 ωt ), is expected to be independent of the CPD and DC bias. To obtain meaningful materials and system properties using conventional KPFM, the dielectric in the tip–sample junction must behave like a lossless dielectric (for example, a vacuum), resulting in both a first harmonic response that is linear with respect to applied DC bias and a time-invariant electrostatic force. At the same time, the measurement itself must not alter the true CPD. These conditions, fundamental to conventional KPFM operation, are expected to be violated in liquids containing mobile ions when AC voltage and/or DC biases are applied due to bias-induced electrochemical and electrokinetic phenomena [17] , [18] , [19] . To date, KPFM has been implemented in liquid in the absence of ions (nonpolar liquid) [20] and limited progress has been obtained in low-molarity electrolytes (<10 mM) using KPFM modes, which do not require bias feedback (for example, open-loop KPFM) [21] , [22] . While electrostatic forces are increasingly being used to actuate atomic force microscope (AFM) cantilever motion in liquids to measure surface topography [23] , [24] , [25] , [26] , surface charge density [26] and dielectric constants [27] , [28] , [29] , voltage-modulated (VM) SPM imaging in conductive electrolytes presents an unresolved challenge. Indeed, in the presence of mobile ions, AC voltage and/or DC bias applied between tip and sample are expected to result in bias-induced charge dynamics, ion diffusion and ultimately Faradaic reactions. These processes alter the force experienced by a VM-SPM probe, precluding meaningful materials and system properties from being obtained using KPFM in the presence of ions, and necessitating the development of a suitable technique to study their influence systematically. Here we establish such a technique paving the way for quantitative, force-based electrochemical measurements in liquid. First, we describe the role mobile ions have on VM-SPM measurements in liquids by modelling the time-dependent ion dynamics for the simplified case of a one-dimensional (1D) parallel-plate capacitor [30] , [31] . We then develop and implement a multidimensional, bias- and time-resolved spectroscopic approach, referred to as electrochemical force microscopy (EcFM). We demonstrate the capability of EcFM to determine CPD under specific conditions and to probe charge screening mechanisms and electrochemical reactions in the probe–sample junction. Finally, we validate EcFM as an imaging mode on a sample with disparate electrochemical properties across its surface. Charging dynamics Recent reports of charge density [26] or electric potential [21] , [22] mapping have been based on the assumption of the presence of a lossless dielectric, and hence a time-invariant electric field in the tip–sample junction. To date, little consideration has been given to the role ion dynamics play on the forces experienced by a VM-SPM probe in liquid. Following the work of refs 10 , 30 , 31 we illustrate the influence of diffuse-charge dynamics on VM-SPM measurements performed in the presence of ions by considering the simple case of a 1D parallel-plate capacitor with ion-blocking electrodes (that is, a non-Faradaic system). We numerically solve the time-dependent ion transport equations using COMSOL Multiphysics and adopting a modified Poisson–Nernst–Plank model [30] , [31] . The model takes into account nonlinear phenomena such as ion diffusion and steric effects including ion crowding, which become particularly important at larger biases (>> kT/e ) and higher ion concentrations. For clarity, we first determine the charge dynamics of the system in response to the application of a small voltage step (30 mV), where steric effects are largely absent ( Fig. 1a ). The electrodes are separated by a distance L =200 nm in a 10 mM 1:1 electrolyte. We observe a time-varying nonlinear potential distribution in the electrode junction. The time it takes the system to reach a steady state (~50 μs, dashed line in Fig. 1a ) can be understood when one considers the relaxation timescales associated with the various electrochemical phenomena involved in reaching electrochemical equilibrium. Once the circuit is closed, ions undergo electromigration in response to the applied electric field, forming electric double layers that electrically screen the polarized electrode. The time it takes an ion to diffuse across the electric double layer is the Debye time, τ D = λ 2 / D , where λ is the Debye screening length and D is the ion diffusivity across λ (ref. 10 ). The Debye time is typically in the ns–μs range for low-molarity aqueous solutions and is 5.2 ns for the model electrolyte capacitor used in Fig. 1a . Even after the formation of the electric double layers, the system has yet to achieve electrochemical equilibrium. The ion concentration gradient away from the electrode surface induces diffusion of ions towards the electrodes, resulting in a net uptake of ions from the neutral bulk electrolyte to the double layer. The timescale of this bulk diffusion process, τ L =( L /2) 2 /D, where L is the electrode separation, is usually much slower (5.7 μs for Fig. 1a ) than the Debye time, as it is governed by the geometry of the system [10] . The third major timescale in the system is the time required for the diffuse layer charge relaxation through bulk electrolyte conduction, τ C =( τ D τ L ) 1/2 = λ ( L /2)/D (172 ns for Fig. 1a ). In equivalent circuit theory, this time is referred to as the electric double-layer charging time (that is, RC time, where R and C are the resistance and capacitance of the circuit). 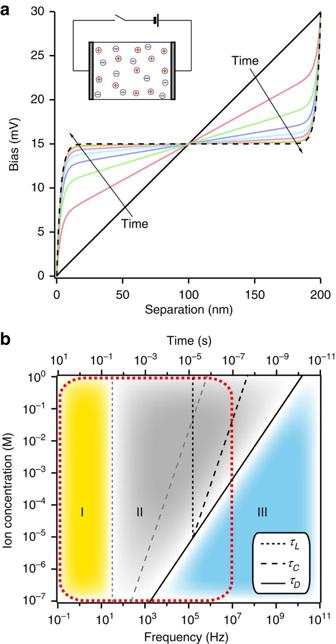Figure 1: Charge dynamics and relaxation processes in the presence of mobile ions. (a) 1D COMSOL model showing the evolution of the bias between plane-parallel electrodes (as shown in the inset) in an 1:1 electrolyte assuming diffusion coefficients,D+=D−=1.77 × 10−9m2s−1(corresponding to the Cl−ion37), with an initial concentration of 10 mM in response to application of a 30 mV voltage step applied across the electrodes (L=200 nm). Solid lines show potential distributions att=0 and then in 100 ns time steps after the bias application. The dashed line shows the distribution att=50 μs after the bias application, which is indistinguishable from the steady-state distribution after the full relaxation of the system. (b) The characteristic timescales (Debye time,τD, bulk diffusion,τL, and charge relaxation,τC) as a function of NaCl concentration for 200 nm (black) and 15 μm (grey) electrode separation representing tip and cantilever samples, respectively. The region enclosed by the red dashed line indicates the frequency space accessible by AFM. The shaded regions indicate the electrochemical processes expected to be present. These relaxation times are calculated for both milliQ water and 10 mM 1:1 electrolyte in Supplementary Table 1 for capacitors with small (200 nm) and large (15 μm) electrode separations, representing the tip- and cantilever-sample distances employed in this work. For larger biases (>30 mV), the picture becomes more complicated due to ion crowding and ultimately Faradaic reactions for non-blocking electrodes. Figure 1: Charge dynamics and relaxation processes in the presence of mobile ions. ( a ) 1D COMSOL model showing the evolution of the bias between plane-parallel electrodes (as shown in the inset) in an 1:1 electrolyte assuming diffusion coefficients, D + = D − =1.77 × 10 −9 m 2 s −1 (corresponding to the Cl − ion 37 ), with an initial concentration of 10 mM in response to application of a 30 mV voltage step applied across the electrodes ( L =200 nm). Solid lines show potential distributions at t =0 and then in 100 ns time steps after the bias application. The dashed line shows the distribution at t =50 μs after the bias application, which is indistinguishable from the steady-state distribution after the full relaxation of the system. ( b ) The characteristic timescales (Debye time, τ D , bulk diffusion, τ L , and charge relaxation, τ C ) as a function of NaCl concentration for 200 nm (black) and 15 μm (grey) electrode separation representing tip and cantilever samples, respectively. The region enclosed by the red dashed line indicates the frequency space accessible by AFM. The shaded regions indicate the electrochemical processes expected to be present. Full size image Diffuse-charge dynamics are present for all tip-sample and cantilever-sample separations, and need to be taken into consideration for all VM-SPM experiments in liquids containing ions. Even under a purely AC voltage excitation, careful consideration must be paid to the timescales of voltage-induced electrochemical processes. Figure 1b shows the evolution of the concentration-dependent ( τ D , τ C ) and -independent ( τ L ) time constants as a function of the calculated relaxation times and ion concentration. The red box indicates the frequency space currently accessible using commercial AFM systems (DC –~10 MHz). Notably, it may be possible to determine the electronic properties (for example, CPD [32] and dielectric constant [27] , [28] ) of the sample when operating in region III, where the electric double-layer charging and ion diffusion processes occur at a timescale much slower than the measurement time (that is, mobile ions are in quasi-static equilibrium) [32] . While measurements of CPD in higher (>100 mM) ion concentrations are attractive for many energy and biological systems, they become impractical in the presence of ion dynamics (region II) and Faradaic processes at longer timescales (region I). At the same time, operating in regions I and/or II presents an opportunity to probe important electrochemical phenomena in the tip–sample junction. These considerations necessitate the development of a multidimensional spectroscopic approach to investigate the role ion dynamics and electrochemical processes play on the forces experienced by a VM-SPM probe. Electrochemical force microscopy The complex time and bias dependences in regions I and II preclude describing ion dynamics in terms of a single parameter (for example, CPD as determined by conventional KPFM). Hence, probing electrochemical phenomena at the solid–liquid interface requires probing bias- and time-resolved dynamics at each spatial point. Here we have developed such a multidimensional spectroscopic approach, referred to as EcFM. In EcFM measurements, the tip is positioned at a specified distance (200 nm for measurements shown) from the surface, and electrochemical processes in the tip–sample junction are activated using a set of bipolar pulses (typically 50–100 ms), amplitude modulated by a slowly varying linear waveform (0.01 Hz). A single-frequency AC excitation ( Fig. 2a ) is used with lock-in detection to record both the amplitude and phase of the first ( A ω and θ ω , respectively) and second (or higher) harmonic responses. The EcFM data are collected both during the bias application (bias-on state) and following the bias application (bias-off state). Here we consider only the bias-on state. In air, the cantilever rapidly responds to the applied bias and quickly reaches, and remains, at equilibrium ( Fig. 2b ). The amplitude response in air has a linear bias dependence, verifying a purely electrostatic response and satisfying key requirements for determining the CPD using conventional KPFM. In liquid, the scenario is more complex and several characteristic bias regimes of dissimilar behaviour are present ( Fig. 2c ). For example, at low biases (<500 mV) the signal shows a relatively weak bias dependence, with small transient processes becoming visible above 200 mV. At larger biases (>500 mV), a relatively strong EcFM response is activated initially, followed by subsequent transient relaxation. Note that the observed nonlinear bias dependence and transient relaxation of the response violate the key requirements for performing conventional KPFM. 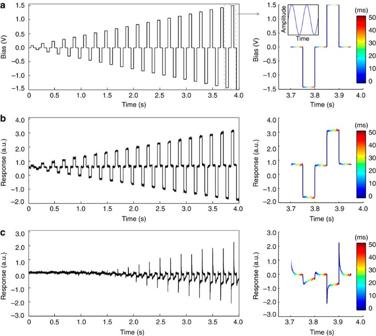Figure 2: Electrochemical force microscopy. (a) Waveform applied to the tip in a single point EcFM measurement. A single-frequency excitation (inset ofa) is applied to the tip, while positive, negative and zero bias pulses are added to the AC voltage. The EcFM response is recorded during both on and off states (measurement window=50 ms) to detect excitation and relaxation processes. Shown is the first harmonic mixed response recorded 200 nm above an Au electrode in (b) air and (c) milliQ water. Figure 2: Electrochemical force microscopy. ( a ) Waveform applied to the tip in a single point EcFM measurement. A single-frequency excitation (inset of a ) is applied to the tip, while positive, negative and zero bias pulses are added to the AC voltage. The EcFM response is recorded during both on and off states (measurement window=50 ms) to detect excitation and relaxation processes. Shown is the first harmonic mixed response recorded 200 nm above an Au electrode in ( b ) air and ( c ) milliQ water. Full size image An alternative illustration of a typical first harmonic EcFM amplitude response is shown in Fig. 3a , where a 2D plot represents the bias and time dependence for a single location, recorded in milliQ water 200 nm above an Au electrode. The maximum in the EcFM amplitude response occurs at <~10 ms, relaxing to an equilibrium value within the measurement window (100 ms). Slight divergence from this equilibrium baseline becomes visible at higher biases (>500 mV). This relatively high response at fast detection rates is comparable to other pulsed electrochemical techniques, where capacitive charging of the electric double layer dominates the response [33] . Similar to KPFM in air, for fast EcFM detection (<1 ms) in milliQ water, we observe a linear bias dependence and amplitude minimum, suggesting that the EcFM response is dominated by an electrostatic interaction (that is, Maxwell stress) in this regime. Under such circumstances, EcFM operation is in principle equivalent to open-loop KPFM operation [34] . The CPD between the tip and Au electrode at 500 μs was determined from a linear fit of the EcFM mixed response (that is, A ω (cos θ ω )) vs bias to be 139±23 mV ( Fig. 3b ). At longer detection times, however, as partial screening of the charge on the electrode occurs, a unique EcFM amplitude minimum is no longer observed, illustrating why the conditions required for conventional KPFM cannot be satisfied in ion-containing solutions ( Supplementary Fig. 1 ). In general, the response was seen to relax to electrochemical equilibrium within 20 ms ( Fig. 3c ), consistent with the disappearance of the amplitude minimum ( Supplementary Fig. 1 ). 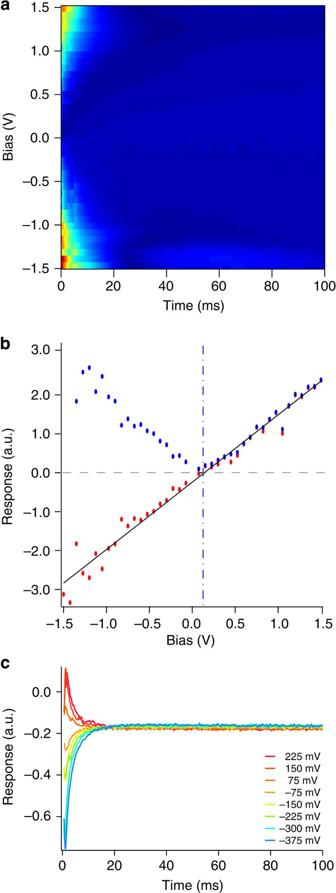Figure 3: Probing charge screening mechanisms using EcFM. (a) 2D plot of the first harmonic EcFM amplitude response 200 nm above the surface. (b) First harmonic EcFM amplitude vs bias (blue data points) and linear fit (black line) to EcFM mixed response (red data points) vs bias dependence for time=500 μs. The CPD, 139±23 mV, is indicated with dashed blue line. (c) EcFM mixed response vs time for a small bias window (−375 to +225 mV). Figure 3: Probing charge screening mechanisms using EcFM. ( a ) 2D plot of the first harmonic EcFM amplitude response 200 nm above the surface. ( b ) First harmonic EcFM amplitude vs bias (blue data points) and linear fit (black line) to EcFM mixed response (red data points) vs bias dependence for time=500 μs. The CPD, 139±23 mV, is indicated with dashed blue line. ( c ) EcFM mixed response vs time for a small bias window (−375 to +225 mV). Full size image Unlike KPFM, EcFM contains important information pertaining to charge screening mechanisms (see Supplementary Figs 2 and 3 ). To demonstrate this, we modelled the charging of polarized capacitor plates separated by 200 nm (tip-sample) and 15 μm (cantilever-sample) in response to a 250 mV bias pulse in milliQ water ( Supplementary Fig. 3 ). Like in any RC circuit, the charging/discharging mechanism of a diffusion-driven process is expected to show a simple exponential decay. In this case, the modelled data were found to be best described by a double exponential fit ( Supplementary Fig. 4 ), with relaxation times of 1.86±0.01 ms and 10.27±0.02 ms. This is in agreement with the experimental data in response to a 225 mV step bias, which yields relaxation time constants of 1.24±0.04 and 6.28±0.21 ms ( Supplementary Fig. 5 ). Note that EcFM data were recorded with bias steps of 75 mV, thus direct comparison with data recorded at 250 mV was not possible. It was also found that for small biases (<10 mV) the modelled electric double layer at a terminal plate demonstrated an exponentially decaying response, whereas for larger biases (>100 mV) a double exponent was required to describe the modelled data ( Supplementary Fig. 4 ). The differences observed between low and high biases are likely a consequence of ion depletion close to the diffuse layers after the electric double-layer screening has occurred. With stronger depletion, the ion redistribution from the bulk will be more noticeable, which is expected for larger biases. In Supplementary Fig. 4 , for all biases investigated, the initial relaxation had a time constant of 1.75±0.10 ms, close to that predicted analytically ( τ C =2.0 ms). For larger biases, a second relaxation process having bias-dependent response times of 3.88±0.07 ms (100 mV) and 10.27±0.05 ms (250 mV) is attributed to the diffusion time of ions from the bulk, τ L =31.8 ms. The bias-dependent deviation between the observed timescales and those determined analytically is not surprising, as the analytical values do not take into account the magnitude of ion depletion and hence have no bias-dependent terms. The osmotic pressure component in our model, which is an indicator of the diffusive processes taking place in the system, also relaxed faster than the diffusion timescale predicted analytically ( τ L =31.8 ms). To explore the dependence of ion concentration on the electrochemical response, EcFM was used to study an Au electrode as a function of K 2 SO 4 concentration ( Fig. 4 ). The first harmonic EcFM amplitude response is represented as response vs bias where each time is represented by a different colour to effectively show the complex bias dependence and subsequent relaxation present within the data. Measurements were performed at 200 nm from the Au surface in milliQ water and 1 mM, 10 mM and 100 mM K 2 SO 4 . In both milliQ water ( Fig. 4a ) and 1 mM K 2 SO 4 ( Fig. 4b ), a bias-dependent response with a minima can be observed in the fast response regime, which quickly relaxes as determined by the RC time of the circuit, τ C . In 1 mM K 2 SO 4 , the transient relaxation time was determined in the same fashion as described for Supplementary Fig. 2a to be 391±90 μs and 1.2±0.1 ms, both of which are beyond the experimental detection limit (limited by the lock-in amplifier time constant, 100 μs). In contrast, for both 10 mM ( Fig. 4c ) and 100 mM K 2 SO 4 ( Fig. 4c ), no significant transient relaxation of the bias dependence in the chosen window (−375 to +225 mV) was observed. The charge screening is expected to occur faster as the concentration increases (2.0 ms for milliQ water and 12.9 μs for 10 mM 1:1 electrolyte, which is well below the current detection limit). To effectively probe charge screening dynamics in higher-molarity electrolytes, sub-microsecond detection [35] could be incorporated into the EcFM setup. Interestingly, at larger biases in high-molarity solutions, we begin to observe a strongly nonlinear response. These processes are too slow (>75 ms) for ion diffusion across the cantilever-sample separation and are attributed to electrochemical reactions taking place at the solid–liquid interfaces. The activation bias of these processes for negative tip bias begins at ~−500 mV for both 10 mM and 100 mM, however, larger amplitudes are observed for 100 mM. Further ion concentration-dependent processes are observed at positive biases (>1.1 V) for 100 mM but not for 10 mM solutions. The concentration dependence of this ‘gap’ between the apparent onset of bias-dependent processes warrants further investigation and requires differentiation of reversible and non-reversible processes. 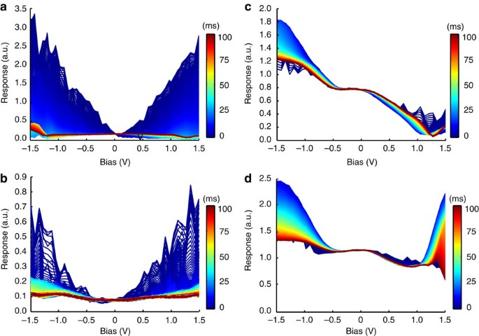Figure 4: EcFM data recorded on Au as a function of ion concentration. The first harmonic EcFM amplitude collected 200 nm above an Au electrode in solutions of increasing salt concentration: (a) milliQ water and (b) 1 mM, (c) 10 mM and (d) 100 mM K2SO4. Measurements were performed from low to high concentrations using the same cantilever. Figure 4: EcFM data recorded on Au as a function of ion concentration. The first harmonic EcFM amplitude collected 200 nm above an Au electrode in solutions of increasing salt concentration: ( a ) milliQ water and ( b ) 1 mM, ( c ) 10 mM and ( d ) 100 mM K 2 SO 4 . Measurements were performed from low to high concentrations using the same cantilever. Full size image Figures 3 and 4 demonstrate that EcFM can be used to investigate charge screening dynamics and electrochemical processes in the probe–sample junction depending on the regime (bias, time, ion concentration). Furthermore, EcFM can be used both to determine CPD and to provide information on charge screening mechanisms. EcFM mapping The EcFM approach allows the 2D bias- and time-dependent spectroscopic responses at a single point to be measured ( Fig. 2 ). The natural question is then whether this strategy can be extended to detect material-specific electrochemical properties and ultimately achieve spatially resolved EcFM imaging, where EcFM response is sampled in a dense spatial grid. Here we introduce such a spectroscopic imaging approach. Shown in Fig. 5 is an example of 2D EcFM imaging in milliQ water across Au electrodes deposited on a SiO 2 layer. Here, 2D EcFM bias- and time-dependent spectroscopic responses were recorded at specified locations in a 30 × 30 grid across the electrodes ( Fig. 5a ), giving rise to a 4D data set ( x , y , bias, time). A quantitative and systematic analysis of the spatial variability of the bias and time dependence of the EcFM response requires a complete physical model of the signal formation mechanism. However, the complexity of the response mechanism in EcFM currently precludes the establishment of a suitable physical model, as is the case for many other AFM techniques (for example, electrochemical strain microscopy). To demonstrate the spatial variability present in the data, we have plotted the first and second harmonic EcFM amplitude responses recorded 5 ms after the onset of the +1.5 and −1.5 V bias pulses ( Fig. 5c–f ). Average cross-sections for each image, from the region indicated in Fig. 5a , are shown in Fig. 5b . The observed spatial variation between Au and SiO 2 is present for all biases and times, as shown in Supplementary Movie 1 . For both first and second harmonics, the EcFM response shows a bias polarity dependence for SiO 2 . This suggests that the effective carrier density of the SiO 2 surface has changed between the application of positive and negative biases. For Au, the first harmonic EcFM response is polarity dependent, whereas the second harmonic response for Au is the same for both ±1.5 V. The presence of such spatially dependent contrast demonstrates that the EcFM signal is localized and dependent on the electrochemical properties of the material below the tip. 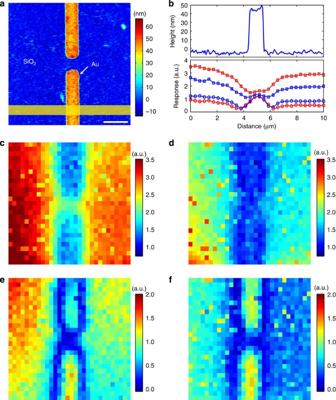Figure 5: Spatial variability of EcFM data recorded across Au/SiO2boundaries in milliQ water. (a) Topography image of Au electrodes on a SiO2substrate recorded using amplitude modulation AFM (scale bar, 2 μm, image size=10 × 10 μm). (b) Average cross-sectional EcFM data recorded 200 nm above the surface and determined from the area marked with a yellow box inafor first (squares) and second (circles) harmonic EcFM amplitude responses during the application of +1.5 V (red) and −1.5 V (blue) bias pulses. Spatial variability maps from a grid of 30 × 30 2D EcFM measurements of the (c,d) first and (e,f) second harmonic EcFM amplitude responses at 5 ms after the onset of the bias-on state for (c,e) +1.5 V and (d,f) −1.5 V, respectively. Figure 5: Spatial variability of EcFM data recorded across Au/SiO 2 boundaries in milliQ water. ( a ) Topography image of Au electrodes on a SiO 2 substrate recorded using amplitude modulation AFM (scale bar, 2 μm, image size=10 × 10 μm). ( b ) Average cross-sectional EcFM data recorded 200 nm above the surface and determined from the area marked with a yellow box in a for first (squares) and second (circles) harmonic EcFM amplitude responses during the application of +1.5 V (red) and −1.5 V (blue) bias pulses. Spatial variability maps from a grid of 30 × 30 2D EcFM measurements of the ( c , d ) first and ( e , f ) second harmonic EcFM amplitude responses at 5 ms after the onset of the bias-on state for ( c , e ) +1.5 V and ( d , f ) −1.5 V, respectively. Full size image We have implemented a generalized approach for electrochemical measurements in liquids containing mobile ions, combining the force sensitivity of AFM with the ability to probe the bias and time dependence of sample-dependent electrochemical dynamics at the probe–sample junction and spatially across boundaries between dissimilar materials. This approach provides a framework to elucidate details of electrochemical processes at the solid–liquid interface. With improvements in detection timescales, EcFM can potentially be used to record and deconvolve fast charge dynamics and electric double-layer formation processes in high-molarity electrolytes. Furthermore, while practical considerations (for example, data acquisition time vs system stability) presently render acquisition of higher-density EcFM images challenging, the adoption of fast lock-in detection and suitable data visualization approaches (for example, principal component analysis [36] ) can make this technique fully viable. EcFM has the potential to provide fundamental insight into ion charge diffusion and relaxation as a function of tip-sample separation and frequency (AC voltage and DC bias sweeps), and may be combined with measurements of current for direct comparison with conventional electrochemical measurements. EcFM measurements will be useful in the study of local electrochemically induced changes in charge density due to both ion adsorption/desorption and electron transfer at the solid–liquid interface and other phenomena central to biological and energy research. Sample preparation Au-coated borosilicate glass substrates (Arrandee) were cleaned in isopropanol and ethanol and rinsed in milliQ water before use. For the Au/SiO 2 sample, ~45 nm of Au was deposited on ~5 nm of Ti by evaporation on top of 100 nm of thermal oxide on Si. EcFM The EcFM measurements were performed using Asylum Research, MFP-3D or Park Systems, NX10 AFM systems, a LabView/MatLab controller implemented using National Instruments NI-5122 and NI-5412 fast AWG and DAQ cards, and as-received Pt/Ir-coated (Nanosensors, PPP-EFM) cantilevers with a nominal mechanical resonant frequency and spring constant of 75 kHz and 2.8 N m −1 , respectively. All measurements were performed using two lock-in amplifiers (Stanford research, SR830 and Signal Recovery, 7280). The time constant of the lock-in amplifiers was set to 100 μs. Excitation frequencies of 17.8 kHz with an amplitude of 1 V were used for Figs 2 , 3 , 4 . For Fig. 5 , the excitation was 19 kHz with an amplitude of 1 V. For Figs 2 and 5 , the DC bias range was ±1.5 V with 50 ms bias-on and -off states, and for Figs 3 and 4 , the DC bias range was ±1.5 V with 100 ms bias-on and -off states. The tip-sample separation was set to 200 nm following a force–distance curve for all EcFM measurements. How to cite this article: Collins, L. et al. Probing charge screening dynamics and electrochemical processes at the solid–liquid interface with electrochemical force microscopy. Nat. Commun. 5:3871 doi: 10.1038/ncomms4871 (2014).